Harvesting dissipated energy with a mesoscopic ratchet The search for new efficient thermoelectric devices converting waste heat into electrical energy is of major importance. The physics of mesoscopic electronic transport offers the possibility to develop a new generation of nanoengines with high efficiency. Here we describe an all-electrical heat engine harvesting and converting dissipated power into an electrical current. Two capacitively coupled mesoscopic conductors realized in a two-dimensional conductor form the hot source and the cold converter of our device. In the former, controlled Joule heating generated by a voltage-biased quantum point contact results in thermal voltage fluctuations. By capacitive coupling the latter creates electric potential fluctuations in a cold chaotic cavity connected to external leads by two quantum point contacts. For unequal quantum point contact transmissions, a net electrical current is observed proportional to the heat produced. In his lectures [1] , Feynman describes a ratchet coupled via an axle to a paddle wheel immersed in a fluid. Because of the Brownian motion of molecules, the paddle wheel has an equal probability to be rotated to the right or the left. Owing to the presence of the pawl preventing one rotation direction, say the left, the ratchet will rotate on the right, seemingly violating the second law of thermodynamics. The apparent contradiction is solved and equal rotation probability restored by including thermal fluctuations of the ratchet. However, if its temperature is smaller than that of the fluid, unidirectional rotation becomes possible, enabling conversion of heat into work. In this letter, we propose a mesoscopic engine composed of two capacitively coupled mesoscopic conductors: a cold and a hot line. To characterize our nanoengine, we separately perform measurements of both hot and cold lines. The temperature increase of the hot line when a bias voltage is applied is measured through Johnson–Nyquist noise of the hot reservoir. Then, we measure the output current of the device and relate it to the temperature difference of both lines ( Supplementary Methods ). We find that the device delivers a net electrical current proportional to the heat produced. Compared with recent realizations on the basis of spin [2] , [3] , superconductors [4] , [5] and graphene [6] , this mesoscopic ratchet device is simple and could be scaled for application in molecular machinery [7] , [8] , [9] . 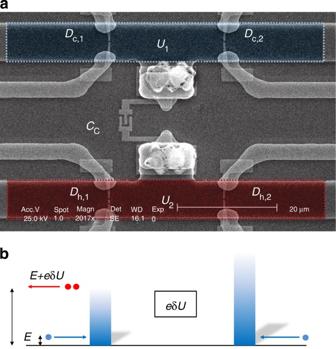Figure 1: Device structure. (a) Scanning electron microscope view of the sample. Two lines defined by wet etching of the mesa are coupled via a coupling capacitanceCC. On the upper line (‘cold’ line) are patterned two QPCs in series (transmissionsDc,1andDc,2) that will define the chaotic cavity (potentialU1). On the lower line (‘hot’ line and potentialU2), a biased QPC enables to heat the line (composed of two QPCs with transmissionsDh,1andDh,2). The metallic capacitance is connected to the cavities via ohmic contacts visible on the picture. (b) Schematic representation of the cold line. Once cold electrons at energyEenter the cavity, they experience voltage fluctuations and gain an energyeδU. Since QPC transmissions are tuned at two different transmissions a net current is generated. Description of the mesoscopic engine Figure 1a shows a scanning electron microscopy picture of our mesoscopic engine, which is on the basis of a proposal described in ref. 10 (the theoretical model is discussed in Supplementary Note 1 ). It consists of two separate ‘cold’ and ‘hot’ circuit lines etched in a high-mobility two-dimensional (2D) electron gas with two quantum point contacts (QPCs) in each ( Supplementary Figs 1 and 2 ). Their temperatures are T 1 and T 2 > T 1 , respectively. The lower line is the heat source: the left QPC is tuned on a conductance plateau and DC-biased in order to generate heat and locally increase the temperature. The series QPC on the right is either tuned on a plateau or opened. To convert the heat into electrical current, it is necessary to define a mesoscopic ratchet together with its mesoscopic pawl. They are implemented in the upper cold circuit line. The ratchet is a chaotic electron cavity defined between two QPCs whose pawl is provided by breaking the symmetry of the energy-dependent transmissions of the left and right QPCs. However, how to convert heat to DC current? A first step is to transfer a part of the thermal voltage fluctuations of the hot circuit into the cold cavity via the coupling capacitance C C . The electrons in the cold cavity are not heated up but their chemical potential experiences a random fluctuation δU , larger than at thermal equilibrium. Then, cold electrons entering the cavity can pick up some fluctuating energy eδU before escaping into the external circuit via the QPCs, see Fig. 1b . If the energy dependence of the transmission of the QPCs is different, one can show that a unidirectional current occurs resulting from the detailed balance of electron flowing in and out the cavity by the left and right ports. In other words, the device generates a net current in the cold line without any applied bias. Figure 1: Device structure. ( a ) Scanning electron microscope view of the sample. Two lines defined by wet etching of the mesa are coupled via a coupling capacitance C C . On the upper line (‘cold’ line) are patterned two QPCs in series (transmissions D c,1 and D c,2 ) that will define the chaotic cavity (potential U 1 ). On the lower line (‘hot’ line and potential U 2 ), a biased QPC enables to heat the line (composed of two QPCs with transmissions D h,1 and D h,2 ). The metallic capacitance is connected to the cavities via ohmic contacts visible on the picture. ( b ) Schematic representation of the cold line. Once cold electrons at energy E enter the cavity, they experience voltage fluctuations and gain an energy eδU . Since QPC transmissions are tuned at two different transmissions a net current is generated. Full size image Measurement of the hot line temperature We now discuss how we proceed to heat the hot circuit and measure its temperature. We apply a DC bias V ds across the left QPC while fixing its transmission D h,1 between 0 and 1. The series QPC is left opened. Joule heating with power is produced on both sides of the QPC within a few electron–electron inelastic scattering lengths, with G = D h,1 2 e 2 / h the QPC conductance ( Supplementary Fig. 3 ). To extract the electronic temperature T e of electrons close to the QPC, we measure the low-frequency current noise. The power spectral density S I is given by [11] : with k B the Boltzmann constant, T e the electronic temperature, G the conductance of the QPC, F the Fano factor defined as F =∑ n D n (1− D n )/∑ n D n ( D n the transmission of the n th channel in the QPC) and − e the charge of the electron. The noise contains information on the electron temperature and on the quantum partitioning of electrons by the QPC, the so-called shot noise. The partition statistics is characterized by the Fano factor, which remarkably goes to zero when the QPC is tuned on a conductance plateau. 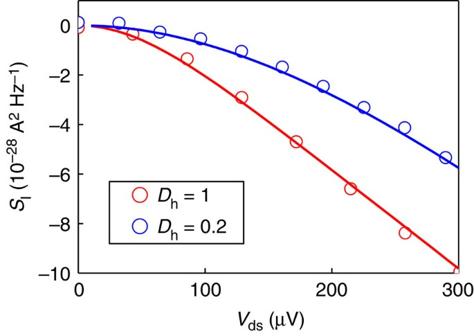Figure 2: Temperature determination. Current noise measurement as a function of the drain source bias for two different QPC transmissionsDhof the hot line. The noise atVds=0 has been subtracted. In blueDh=1, in redDh=0.2 (a feedback loop on the measured differential conductance ensures the stability of transmissions). At small bias, a QPC tuned on a plateau is noiseless. However, at larger bias, the dissipated power combined with the Wiedemann–Franz law implies an elevation of the temperature and a larger Johnson–Nyquist noise (black dotted line). The experimental values are well fitted when considering all three possible thermal anchors (blue solid line). ForDh=0.2, we need to consider both usual shot noise together with this additional heating (red solid line). Figure 2 shows the excess shot noise measurements (we subtract the zero bias shot) as a function of V ds for two different transmissions D 1 = D h,1 =0.2 and 1. For D h,1 =0.2, we observe the partitioning noise as expected. On a conductance plateau the second term of equation 1, corresponding to shot-noise, is zero. The excess noise is only due to equilibrium thermal noise or Johnson–Nyquist noise: S I ( V ds )=4 k B T e ( V ds ) G . The non-zero value of the noise corresponds to the increase in Johnson–Nyquist noise as function of the bias. The increase in electronic temperature with Joule heating power is accurately described using the Wiedemann–Franz law of electron thermal conduction ( Supplementary Note 2 ). This is applicable here as the gradient of electronic temperature T e from the QPC to base temperature at the ohmic contacts, occurs on a length of the order of the electron–phonon energy relaxation length. Combining the Joule power with the Wiedemann–Franz law, we expect [12] , [13] : Figure 2: Temperature determination. Current noise measurement as a function of the drain source bias for two different QPC transmissions D h of the hot line. The noise at V ds =0 has been subtracted. In blue D h =1, in red D h =0.2 (a feedback loop on the measured differential conductance ensures the stability of transmissions). At small bias, a QPC tuned on a plateau is noiseless. However, at larger bias, the dissipated power combined with the Wiedemann–Franz law implies an elevation of the temperature and a larger Johnson–Nyquist noise (black dotted line). The experimental values are well fitted when considering all three possible thermal anchors (blue solid line). For D h =0.2, we need to consider both usual shot noise together with this additional heating (red solid line). Full size image with G m the total conductance linking the QPC to the ohmic contacts and T fridge the base temperature. In practical, we have to consider the cooling effect of the inner ohmic contact (see Supplementary Note 2 ). Within this approach, we explain our measurements for D h,1 =0.2 (red solid line in Fig. 2 ) and on the plateau (blue solid line in Fig. 2 ). Typically, for an applied bias of 1 mV and D h,1 =1, we get Δ T = T 2 − T 1 =806 mK. Conversion of heat to current We next investigate conversion of heat to current. A necessary condition to generate a net current is to create an asymmetry between the two QPCs of the cold circuit line. In a first experiment, we have tuned the second QPC at D c,2 =0.5 and have swept the first QPC transmission D c,1 between 0 and 2. To ensure the highest temperature difference Δ T between the two lines, both QPCs of the hot line are tuned on the first plateau (in fact the second QPC shows no good conductance plateau, which may generate a small additional noise). Then, we increase by steps of ~1 mV the applied bias V ds while sweeping the transmission. The different traces of Fig. 3a show that the absolute value of the current increases with V ds . It is zero when the transmission D c,1 ~0.75, that is, when the detailed balance of input/output electrons is symmetrical. Then, the current changes sign as expected when the symmetry of the cavity is reversed, a hallmark of the ratchet effect. To model the current variation and have a quantitative understanding of the ratchet effect, we follow the semiclassical approach developed by Sothmann et al. [10] . 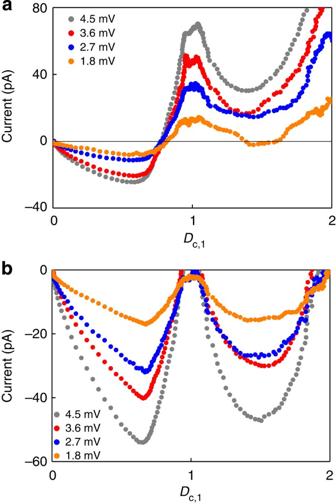Figure 3: Harvested current. (a) Both QPCs of the hot line are tuned on a plateau (Dh,1=1 andDh,2=1). Current measured in the cold line as a function of the first QPC transmissionDc,1forDc,2=0.5 for applied bias voltages from 1.8 to 4.6 mV. WhenDc,1~0.5, the symmetry of the cavity is reversed and the sign of the current changes. (b) Both QPCs of the hot line are tuned on a plateau (Dh,1=1 andDh,2=1). Current measured in the cold line as a function of the first QPC transmissionDc,1forDc,2=1. When temperature difference ΔTbetween the two lines is increased by applying a larger bias on the hot line, the current is enhanced. We sweep the applied bias from 1.8 to 4.6 mV. Considering the symmetry-breaking in the energy derivatives of the transmissions of the cold line, the authors find a DC current generated by heat conversion in the cold line given by: Figure 3: Harvested current. ( a ) Both QPCs of the hot line are tuned on a plateau ( D h,1 =1 and D h,2 =1). Current measured in the cold line as a function of the first QPC transmission D c,1 for D c,2 =0.5 for applied bias voltages from 1.8 to 4.6 mV. When D c,1 ~0.5, the symmetry of the cavity is reversed and the sign of the current changes. ( b ) Both QPCs of the hot line are tuned on a plateau ( D h,1 =1 and D h,2 =1). Current measured in the cold line as a function of the first QPC transmission D c,1 for D c,2 =1. When temperature difference Δ T between the two lines is increased by applying a larger bias on the hot line, the current is enhanced. We sweep the applied bias from 1.8 to 4.6 mV. Full size image with Λ a rectification parameter, characterizing the asymmetry (the ratchet): where G c, i =( e 2 / h ) D c, i , (with the derivative as a function of the energy ) and G c,Σ the total conductance in parallel for the cold line. We introduce G eff an effective conductance of the double cavity, G eff = G c,Σ G h,Σ /( G c,Σ + G h,Σ ) ( G c,Σ = G c,1 + G c,2 , same for G h,Σ ) and C eff that grows as (a complete description of C eff is given in Supplementary Note 1 ) and takes into account the various capacitive couplings of the device. For a good electrical energy-harvesting, C eff has to be minimized. is an effective RC time of the double cavity. In Fig. 3a we tune D c,2 ~0.5 and in Fig. 3b D c,2 ~1. In the first case, the derivative of D c,2 is non-zero, and we would expect a change of the current sign around D c,1 ~0.5 if both QPCs were identical, it appears instead around D c,1 ~0.75 because of QPCs’ asymmetry. In the second one, the derivative is zero and we should not have a change of the current sign in agreement with our measurements. In both cases, we check that by increasing the bias, we indeed enhance Δ T and measure a larger current. We now discuss the measured current compared with the expected values. We consider the case where D h,2 ~1. Since both QPCs are now tuned on a plateau, the temperature calculation is slightly different from equation (2) ( Supplementary Fig. 4 and Supplementary Note 2 ). For 1 mV applied on QPCs, we get Δ T ~2.5 K. As expected, the temperature difference is larger when the series QPC is tuned on the first plateau compared with the opened case. To obtain , one follows the saddle point model of a QPC [14] where the transmission of the n th mode can be written where ω n , x is related to the negative curvature of the saddle point potential (see Supplementary Note 1 ). The lever arm is extracted from transconductance (d G c, i /d V g ) measurements Δ~0.02 e . C eff is given by the geometry of the device. C C =1 fF and C μ =C Σ =5 fF are realistic values confirmed by electrostatic simulations, giving C eff =105 fF. Finally, we extract I c ~20 pA for D c,1 =0.5 and an applied bias of 1.8 mV, in agreement with measurements. In this last part, we aim to proceed to a complete mapping of the current as a function of the two barriers of the cold line and to compare it with the theory. To do this, we apply a 2-mV DC bias on the hot line, we tune the first QPC on its first plateau while opening the second QPC (doing this we make sure that we remain on the first plateau, exclude any additional source of noise as partition noise). Measurements are plotted in Fig. 4a . Since the second QPC of the hot line is opened, current fluctuations are reduced compared with the previous configuration and the current is smaller compared with Fig. 3a (the current is at the limit of the detection set-up sensitivity, which causes the apparent inhomogeneity of the current map). As expected, the current is zero when barrier transmissions are equal and maximum for the most asymmetric configuration. We also check that the sign of the current changes when the role of the transmission is reversed. We compare these measurements with theoretical predictions in Fig. 4b . We observe a good qualitative agreement with our data taking C eff ~0.4 pF, an increase attributed to the opened series QPC in the hot line and a much bigger cavity. 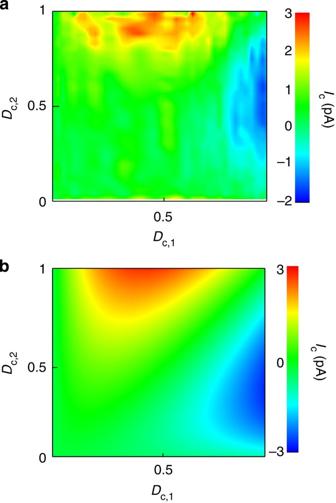Figure 4: Current map. (a) Colour plot of the current measured in the cold line as a function of the first QPC transmissionDc,1(xaxis) and the second oneDc,2(yaxis). The applied bias on the hot line is equal to 2 mV. The first QPC of the hot line is tuned on the first plateau, although the series QPC is opened. When the symmetry of the barriers is inverted the sign of the current changes. (b) Expected current as a function of bothDc,1andDc,2forCeff~0.4 pF. We recover experimental features, as a zero current along the lineDc,1=Dc,2, and a reverse current when the symmetry of the barriers is changed. Figure 4: Current map. ( a ) Colour plot of the current measured in the cold line as a function of the first QPC transmission D c,1 ( x axis) and the second one D c,2 ( y axis). The applied bias on the hot line is equal to 2 mV. The first QPC of the hot line is tuned on the first plateau, although the series QPC is opened. When the symmetry of the barriers is inverted the sign of the current changes. ( b ) Expected current as a function of both D c,1 and D c,2 for C eff ~0.4 pF. We recover experimental features, as a zero current along the line D c,1 = D c,2 , and a reverse current when the symmetry of the barriers is changed. Full size image We have realized a mesoscopic Brownian ratchet. A ‘hot’ cavity is capacitively coupled to a ‘cold’ mesoscopic ratchet composed of two QPCs in series. Depending on the symmetry of these two barriers, a current can be measured in the cold line. We have fully mapped the current as a function of these two barrier transmissions, in agreement with theoretical predictions. This set-up is a prototype of a mesoscopic engine that would harvest dissipated energy, transforming it into electrical current. In this heat engine device, the energy-harvesting efficiency is low η =5 × 10 −5 (detailed calculations in Supplementary Note 3 ); however, there is still a lot of room for improvement. First, self-capacitances to the ground should be lowered: this can be performed by reducing the area of the cavity. Precise calculations of the electrostatic environment will determine the optimal capacitance C C that will minimize the parameter C eff . Among the different thermoelectric heat engines [15] , [16] , [17] , [18] , [19] , [20] , a considerable advantage of our heat engine is the absence of direct electrical connection between hot and cold sources. This suppresses electron thermal conduction and thus reduces the thermal shunt between hot and cold sources. The two reservoirs are coupled via an electric capacitance, and only phonons can provide a thermal shunt between them. Therefore, this system is suitable when electrical isolation is an issue for applications, as there is not direct electrical connection between hot and cold sources. After optimization, the mesoscopic energy-harvesting engine may solve the heat-removal problem. Sample fabrication and experimental set-up Emitter and detector lines were patterned using e-beam lithography on a high-mobility two-dimensional electron gas formed at the GaAs/Ga 1− x Al x As heterojunction. The two-dimensional electron gas 100 nm below the surface has a density of 1.8 × 10 11 cm −2 and mobility 2.69 × 10 6 cm 2 V −1 s −1 . Measurements were performed in cryogen-free 3 He cryostat with 300-mK base temperature (more details in Supplementary Methods ). To elevate the electronic temperature of the hot line a finite V dc is applied on the upper line. The resulting voltage fluctuations induce a photocurrent I ph in the detector. We pulse V dc at 1.5 kHz and detect the induced photocurrent using a lock-in technique. How to cite this article: Roche, B. et al. Harvesting dissipated energy with a mesoscopic ratchet. Nat. Commun. 6:6738 doi: 10.1038/ncomms7738 (2015).